Soluble forms of polyQ-expanded huntingtin rather than large aggregates cause endoplasmic reticulum stress In Huntington’s disease, as in other neurodegenerative diseases, it was initially thought that insoluble protein aggregates are the toxic species. However, growing evidence implicates soluble oligomeric polyglutamine-expanded huntingtin in cytotoxicity. Here we show that pathogenic huntingtin inhibits endoplasmic reticulum (ER)-associated degradation and induces ER stress before its aggregation into visible inclusions. All three branches of the unfolded protein response are activated. ER stress can be compensated by overexpression of p97/VCP, suggesting its sequestration by pathogenic huntingtin as a main cause. Stress correlates with the presence of huntingtin oligomers and is independent of continual huntingtin synthesis. Stress levels, measured in striatal neurons, are stabilized but only slowly subside on huntingtin aggregation into inclusions. Our results can be explained by the constant conversion of huntingtin monomers to toxic oligomers; large aggregates sequester the former, precluding further conversion, whereas pre-existing toxic oligomers are only gradually depleted. Huntington’s disease (HD) is a neurodegenerative disorder arising from an expanded polyglutamine (polyQ) tract (>35 amino acids) in the huntingtin (Htt) protein. This mutation causes Htt aggregation, interfering in several ways with normal cell metabolism [1] , [2] , [3] and leading to cell death through a not yet elucidated mechanism. Especially affected in HD are cells of the brain striatum [4] . One of the pathways affected by mutant Htt is the ubiquitin-proteasome system (UPS) [5] , [6] . Interference with the UPS inhibits cytosolic protein degradation as well as endoplasmic reticulum (ER)-associated protein degradation (ERAD) [7] , [8] , a pathway that reduces the protein load in the ER [9] , [10] . Inhibition of ERAD leads to the accumulation of unfolded or misfolded proteins in the ER, ER stress and the activation of the unfolded protein response (UPR) [7] , [11] , [12] , (reviewed in refs 13 , 14 ). There is increasing evidence that Htt oligomers and not aggregates are the cytotoxic agent in HD [3] , [15] , [16] , although the subject still remains controversial. PolyQ-expanded Htt has been reported to inhibit the UPS before its inclusion into large aggregates [17] , [18] , which prompted us to analyse whether the generation of ER stress, with its long-term cytotoxic effects, is an early or late event. Here we analysed the effect of pathogenic Htt on ERAD and UPR activation, focusing on the role of its aggregation in the process. We present unambiguous evidence that inhibition of ERAD and induction of ER stress occur before appearance of visible aggregates. PolyQ-expanded Htt slows ERAD and causes ER stress We tested the effect of polyQ-expanded Htt on an established ERAD substrate, uncleaved precursor of asialoglycoprotein receptor H2a. Endogenously expressed in hepatocytes, H2a membrane precursor undergoes cleavage to a secreted form, but when expressed in other cell types, cleavage is inefficient and the protein is degraded by the UPS [19] , [20] . The ERAD substrate accumulated when expressed in HEK 293 cells in the presence of Htt96Q (containing exon 1 with an expanded tract of 96 glutamines; Fig. 1a ). Also in striatal cells (those most relevant to HD), pulse-chase analysis indicated that degradation of the ERAD substrate was strongly inhibited by coexpression of Htt96Q relative to Htt20Q (a non-pathogenic form; Fig. 1b ). An early response to proteasomal inhibition or ER stress is the accumulation of ERAD substrate proteins, chaperones and components of the UPR and ERAD machineries in the juxtanuclear ER-derived quality control compartment (ERQC), a putative staging ground for ERAD [19] , [21] . Htt96Q caused a strong ERQC accumulation of H2a-RFP or H2a–green fluorescent protein (GFP) fusion proteins and of endogenous calnexin ( Fig. 1c,d and Fig. 2 ), whereas there was no effect of Htt20Q. The effect of Htt96Q was especially strong in striatal neurons compared with other cell types ( Fig. 3 ). As we had seen before, proteasomal inhibition did not cause accumulation of the ER chaperone BiP in the ERQC ( Fig. 2a ), it remained in an ER pattern also on Htt96Q expression ( Fig. 3d ). We observed that H2a and calnexin accumulation occurred in most cells containing large Htt96Q inclusions and not when Htt was in a diffuse, apparently non-aggregated pattern in the cytosol or the nucleus ( Figs 1c,d , 2 and 3 ). The cellular localization of the Htt96Q large inclusion bodies varied and was unrelated to the localization of the accumulated H2a-RFP ( Fig. 3 ). 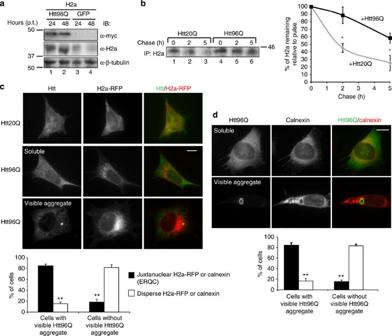Figure 1: PolyQ-expanded Htt inhibits ERAD and causes protein and chaperone accumulation in the ERQC. (a) The ERAD substrate H2a accumulates in HEK 293 cells expressing myc-tagged Htt96Q, but not in the control GFP-expressing cells. Post-transfection (p.t.) times are indicated. Blots representative of three independent experiments are shown. (b) Inhibition of H2a degradation on expression of Htt96Q, but not of Htt20Q is revealed by metabolic labelling with [35S]-cysteine in striatal STHdhQ7/7cells. The graph shows percent of H2a in the chase relative to pulse (100%), as an average of three experiments±s.e. (*P-value 2 h=0.03, *P-value 5 h=0.05, Student’st-test (unpaired, two-tailed)). The experiments were performed with Htt containing only exon 1 of a polyQ-expanded Htt, a commonly used model that recapitulates the aggregation-prone behaviour of the whole protein34,35. Coexpression of Htt7Q in the striatal cells mimics the typical heterozygous expression of pathogenic Htt from one allele in HD patients. (c,d) Very strong accumulation of H2a-RFP (c) and of calnexin (d) in the ERQC in STHdhQ7/7cells, apparently correlated to Htt96Q-myc visible aggregate formation. Htt20Q-myc does not affect the distribution of H2a-RFP in the ER (c). Scale bar, 10 μm. The graphs show the percent of cells with H2a-RFP (c) or calnexin (d) accumulated in the juxtanuclear region (ERQC, black bars) and those showing a disperse ER pattern (white bars) in STHdhQ7/7cells with visibly aggregated versus soluble Htt96Q. Bars are averages of three independent experiments±s.e. (N>60 in each) (**P-value<0.005, Student’st-test (unpaired, two-tailed)). Figure 1: PolyQ-expanded Htt inhibits ERAD and causes protein and chaperone accumulation in the ERQC. ( a ) The ERAD substrate H2a accumulates in HEK 293 cells expressing myc-tagged Htt96Q, but not in the control GFP-expressing cells. Post-transfection (p.t.) times are indicated. Blots representative of three independent experiments are shown. ( b ) Inhibition of H2a degradation on expression of Htt96Q, but not of Htt20Q is revealed by metabolic labelling with [ 35 S]-cysteine in striatal ST Hdh Q7/7 cells. The graph shows percent of H2a in the chase relative to pulse (100%), as an average of three experiments±s.e. (* P -value 2 h=0.03, * P -value 5 h=0.05, Student’s t -test (unpaired, two-tailed)). The experiments were performed with Htt containing only exon 1 of a polyQ-expanded Htt, a commonly used model that recapitulates the aggregation-prone behaviour of the whole protein [34] , [35] . Coexpression of Htt7Q in the striatal cells mimics the typical heterozygous expression of pathogenic Htt from one allele in HD patients. ( c , d ) Very strong accumulation of H2a-RFP ( c ) and of calnexin ( d ) in the ERQC in ST Hdh Q7/7 cells, apparently correlated to Htt96Q-myc visible aggregate formation. Htt20Q-myc does not affect the distribution of H2a-RFP in the ER ( c ). Scale bar, 10 μm. The graphs show the percent of cells with H2a-RFP ( c ) or calnexin ( d ) accumulated in the juxtanuclear region (ERQC, black bars) and those showing a disperse ER pattern (white bars) in ST Hdh Q7/7 cells with visibly aggregated versus soluble Htt96Q. Bars are averages of three independent experiments±s.e. ( N >60 in each) (** P -value<0.005, Student’s t -test (unpaired, two-tailed)). 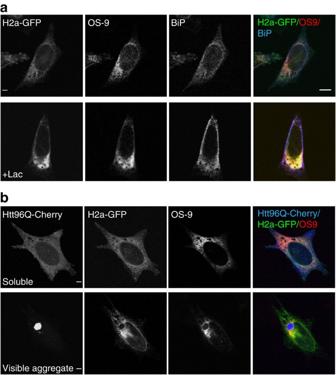Figure 2: ERAD substrate accumulation in the ERQC on proteasomal inhibition or expression of pathogenic Htt. (a) STHdhQ7/7cells show localization of OS-9 in the ERQC both in untreated and in proteasome-inhibited cells (+Lac), whereas H2a accumulates in the compartment only under stressed conditions. BiP remains disperse through the peripheral ER both in normal and stressed conditions. Scale bar, 10 μm. (b) H2a-RFP accumulation as inFig. 1c, but including S-tagged OS-9 as a marker of the ERQC, where H2a accumulates during the Htt96Q aggregate formation. The cells were grown for 24 h after transfection before fixation in all cases. Full size image Figure 2: ERAD substrate accumulation in the ERQC on proteasomal inhibition or expression of pathogenic Htt. ( a ) STHdh Q7/7 cells show localization of OS-9 in the ERQC both in untreated and in proteasome-inhibited cells (+Lac), whereas H2a accumulates in the compartment only under stressed conditions. BiP remains disperse through the peripheral ER both in normal and stressed conditions. Scale bar, 10 μm. ( b ) H2a-RFP accumulation as in Fig. 1c , but including S-tagged OS-9 as a marker of the ERQC, where H2a accumulates during the Htt96Q aggregate formation. The cells were grown for 24 h after transfection before fixation in all cases. 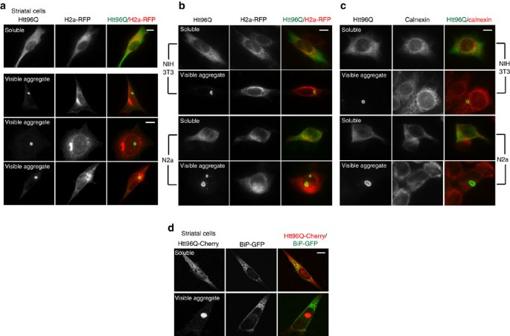Figure 3: Strong accumulation of H2a and calnexin in the ERQC in the presence of visible Htt96Q aggregates in striatal neurons. (a) The localization of H2a accumulation is not correlated with Htt96Q aggregate localization. Similar to the experiment inFig. 1c. (b,c) Non-striatal cells are less affected by large Htt96Q aggregates. Similar to the experiments inFig. 1c,d, but with NIH 3T3 and N2a cells. (d) As ina, but with BiP-GFP expression and Htt96Q-Cherry. Htt96Q aggregation does not affect the disperse pattern of BiP-GFP through the ER. Scale bar, 10 μm in all panels. Full size image Figure 3: Strong accumulation of H2a and calnexin in the ERQC in the presence of visible Htt96Q aggregates in striatal neurons. ( a ) The localization of H2a accumulation is not correlated with Htt96Q aggregate localization. Similar to the experiment in Fig. 1c . ( b , c ) Non-striatal cells are less affected by large Htt96Q aggregates. Similar to the experiments in Fig. 1c,d , but with NIH 3T3 and N2a cells. ( d ) As in a , but with BiP-GFP expression and Htt96Q-Cherry. Htt96Q aggregation does not affect the disperse pattern of BiP-GFP through the ER. Scale bar, 10 μm in all panels. Full size image The observed accumulation of the ERAD substrate could be an early sign of ER stress. Indeed, all three branches of the UPR, the PERK, ATF6 and IRE1 pathways [22] , were activated by expression of Htt96Q in a time-dependent manner and in correlation with the presence of insoluble Htt96Q aggregates ( Fig. 4 ). The activation of the IRE1 pathway was also confirmed in individual cells by using an XBP1-venus reporter protein [23] . This protein is not fluorescent when in its full-length unspliced form. Splicing by activated IRE1 allows venus into its correct open reading frame, producing a fluorescent protein. XBP1-venus was spliced and showed a fluorescent signal in cells with Htt96Q aggregates, but not in cells expressing Htt20Q ( Fig. 4d ). 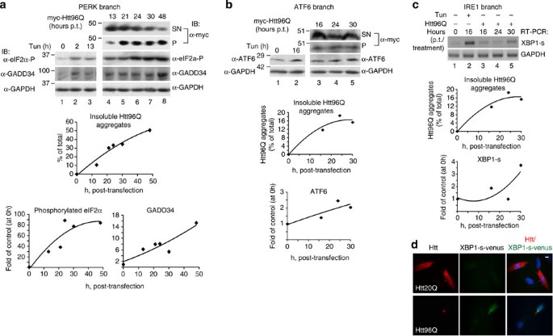Figure 4: Induction of all three UPR branches by Htt96Q seems to correlate with insoluble aggregate formation. (a,b) Increase in phosphorylated eIF2α, GADD34 (a, PERK branch of the UPR) and ATF6 fragment levels (b) correlate with the accumulation of Htt96Q insoluble aggregates (P, pellet) over time, and not with its soluble fraction (SN, supernatant) in HEK 293 cells. (c) Spliced XBP1 mRNA levels (XBP1-s, IRE1 branch of the UPR) measured by RT–PCR analysis of parallel samples of the experiment inbalso increase with Htt96Q aggregation. Tunicamycin (Tun, 5 μg ml−1) was used as a positive control for UPR induction. Values were corrected by GAPDH protein (a,b) or RT–PCR (c) as the loading control. (d) Splicing of XBP1-venus apparently correlates with the presence of large Htt96Q aggregates. XBP1-venus reporter protein, lacking its DNA-binding domain, was expressed together with myc-tagged Htt20Q or Htt96Q in STHdhQ7/7cells. Cells were fixed and stained with anti-myc. Splicing of XBP1-venus mRNA brings venus into its correct open reading frame, producing a fluorescent protein. The fluorescence appears in Htt96Q- but not in Htt20Q-expressing cells. Scale bar, 10 μm. Figure 4: Induction of all three UPR branches by Htt96Q seems to correlate with insoluble aggregate formation. ( a , b ) Increase in phosphorylated eIF2α, GADD34 (a, PERK branch of the UPR) and ATF6 fragment levels ( b ) correlate with the accumulation of Htt96Q insoluble aggregates (P, pellet) over time, and not with its soluble fraction (SN, supernatant) in HEK 293 cells. ( c ) Spliced XBP1 mRNA levels (XBP1-s, IRE1 branch of the UPR) measured by RT–PCR analysis of parallel samples of the experiment in b also increase with Htt96Q aggregation. Tunicamycin (Tun, 5 μg ml −1 ) was used as a positive control for UPR induction. Values were corrected by GAPDH protein ( a , b ) or RT–PCR ( c ) as the loading control. ( d ) Splicing of XBP1-venus apparently correlates with the presence of large Htt96Q aggregates. XBP1-venus reporter protein, lacking its DNA-binding domain, was expressed together with myc-tagged Htt20Q or Htt96Q in STHdh Q7/7 cells. Cells were fixed and stained with anti-myc. Splicing of XBP1-venus mRNA brings venus into its correct open reading frame, producing a fluorescent protein. The fluorescence appears in Htt96Q- but not in Htt20Q-expressing cells. Scale bar, 10 μm. Full size image ER stress correlates with presence of mutant Htt oligomers The above experiments suggested inhibition of ERAD and induction of ER stress correlating with the formation of visible and insoluble Htt aggregates. However, those experiments did not resolve the formation of large aggregates from that of soluble intermediate Htt oligomers. It had been reported before that expression of pathogenic Htt causes ER stress [7] , [11] , [12] , but the molecular form of Htt that causes this effect had not been determined. On the other hand, there is increasing evidence that Htt oligomers and not aggregates are the cytotoxic agent [3] , [15] , [16] , although it is not clear what cellular pathways they affect. Therefore, we analysed the activation of the UPR pathways in conditions that allowed us to resolve soluble oligomeric Htt96Q from insoluble aggregates. This was done by using an inducible TEToff system, where we could shut off Htt96Q synthesis using doxycycline (Dox) and follow the presence of oligomers, insoluble aggregates and UPR markers with time [3] . The fraction of Htt96Q in oligomers in cell extracts reached its peak 48 h after transfection (24 h without Dox followed by 24 h with Dox), when oligomers were more abundant than insoluble aggregates ( Fig. 5a,b,d ). Oligomers were fractionated by centrifugation through glycerol gradients after separation from insoluble aggregates (Methods) and showed a broad range of molecular weight, peaking around 300 kDa ( Fig. 5a , 48 h). Interestingly, Htt fragments present in oligomers at 40–48 h were smaller in size than those in monomers, having probably undergone a proteolytic cleavage after or immediately before oligomerization. At 54 h after transfection (30 h without Dox followed by 24 h with Dox), insoluble aggregates were abundant ( Fig. 5b ), whereas oligomers were at a minimum ( Fig. 5a ). The phosphorylated form of translation factor eIF2α, an early UPR marker, showed a low level in the presence of Dox, increasing slowly with time; its levels peaked at early times in the absence of Dox (24 h after transfection), coinciding with the initial appearance of oligomeric forms ( Fig. 5a,b ). The levels of the UPR markers BiP, XBP1-s and GADD34 correlated with the presence of oligomers and not insoluble aggregates ( Fig. 5b–e ). Whereas the fraction of Htt in insoluble aggregates increased from 48 to 54 h, the levels of these UPR markers decreased between those time points. These results suggest that Htt96Q oligomers and not large insoluble aggregates are the inducers of ER stress. 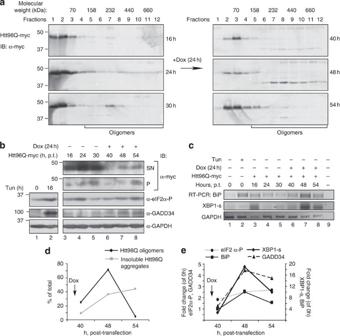Figure 5: Temporal resolution of Htt96Q oligomeric forms and insoluble aggregates shows correlation of UPR induction with the presence of oligomers (a–c). Parallel samples of HEK 293 cells expressing myc-tagged Htt96Q for 16, 24 or 30 h were incubated with Dox (1 μg ml−1) for another 24 h (40, 48 and 54 h, respectively). The soluble fraction of a larger amount of each sample (60% of total) was fractionated in glycerol gradients (a). Smaller amounts (20% of total) were subjected to protein (b) and mRNA (c) detection. Fractions 5–12 inaare defined as oligomers (Htt96Q monomer is around 50 kDa). P=pellet (insoluble aggregates) and SN=supernatant (monomers+oligomers) inb. Overnight treatment with tunicamycin (5 μg ml−1,b,c) was used as a positive control for UPR induction. Values were corrected by GAPDH levels, used as a loading control as inFig. 4. (d,e) The graphs summarize the results presented ina–c. SN+P inbcorresponds to total Htt at each time point. Percent of total Htt was P × 100/(SN+P) for insoluble aggregates and for oligomers it was oligomers × 100/total (SN) at each time point inamultiplied by SN × 100/(SN+P) inband divided by 100; the remainders are monomers (not plotted). Especially informative are time points of 48 h, when oligomers are preponderant, and 54 h, when there are insoluble aggregates but almost no oligomers. Increase in BiP, XBP1-s and GADD34 levels correlates with the accumulation of Htt96Q oligomers. Shown is a representative of three experiments. Figure 5: Temporal resolution of Htt96Q oligomeric forms and insoluble aggregates shows correlation of UPR induction with the presence of oligomers ( a – c ). Parallel samples of HEK 293 cells expressing myc-tagged Htt96Q for 16, 24 or 30 h were incubated with Dox (1 μg ml −1 ) for another 24 h (40, 48 and 54 h, respectively). The soluble fraction of a larger amount of each sample (60% of total) was fractionated in glycerol gradients ( a ). Smaller amounts (20% of total) were subjected to protein ( b ) and mRNA ( c ) detection. Fractions 5–12 in a are defined as oligomers (Htt96Q monomer is around 50 kDa). P=pellet (insoluble aggregates) and SN=supernatant (monomers+oligomers) in b . Overnight treatment with tunicamycin (5 μg ml −1 , b , c ) was used as a positive control for UPR induction. Values were corrected by GAPDH levels, used as a loading control as in Fig. 4 . ( d , e ) The graphs summarize the results presented in a – c . SN+P in b corresponds to total Htt at each time point. Percent of total Htt was P × 100/(SN+P) for insoluble aggregates and for oligomers it was oligomers × 100/total (SN) at each time point in a multiplied by SN × 100/(SN+P) in b and divided by 100; the remainders are monomers (not plotted). Especially informative are time points of 48 h, when oligomers are preponderant, and 54 h, when there are insoluble aggregates but almost no oligomers. Increase in BiP, XBP1-s and GADD34 levels correlates with the accumulation of Htt96Q oligomers. Shown is a representative of three experiments. Full size image P97/VCP can compensate the ERAD inhibition and ER stress We next searched for a possible cause of this ER stress induction. One protein that is important for ERAD and was shown to be sequestered in Htt aggregates is the AAA ATPase and cytosolic chaperone p97/VCP (refs 7 , 24 ). Overexpression of p97 caused a pronounced reduction in eIF2α phosphorylation at early times of Htt96Q expression ( Fig. 6a ), apparently without affecting Htt96Q levels, suggesting a compensatory effect for p97 sequestration. P97 had only a very minor effect in reducing the aggregation of Htt96Q ( Fig. 6b ). P97 did alleviate significantly the accumulation of the ERAD substrate, H2a, caused by Htt96Q expression ( Fig. 6b ). The inhibition of H2a degradation on Htt96Q expression was suppressed by p97 overexpression ( Fig. 6c ). 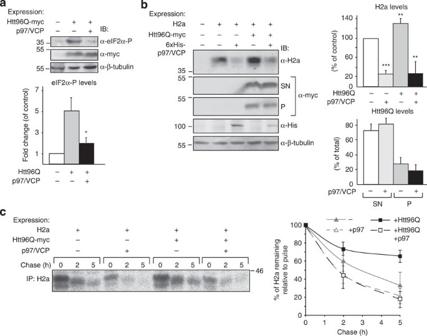Figure 6: ERAD inhibition and ER stress triggered by Htt96Q can be compensated by overexpression of p97/VCP. (a) Induction of eIF2α phosphorylation after 24 h of Htt96Q expression is strongly inhibited by coexpression of p97/VCP. (*P-value=0.02, Student’st-test (unpaired, two-tailed)). (b) Accumulation of H2a caused by Htt96Q expression is strongly reduced by coexpression of p97/VCP. P97/VCP has only a minor, non-significant effect in reducing the Htt96Q fraction in insoluble aggregates. Values were corrected by the anti-β-tubulin signal as a loading control. (**P-value<0.01, ***P-value=0.00006, Student’st-test (unpaired, two-tailed)). (c) Inhibition of H2a degradation on expression of Htt96Q is cancelled by overexpression of p97/VCP. Experiment similar to that inFig. 1bbut in HEK 293 cells with and without coexpression of p97. The graph shows percent of H2a in the chase relative to pulse (100%). Where indicated, p97 overexpression was done using 6xHis-tagged p97/VCP in all cases. All graphs in this figure are averages of three experiments±s.e. Figure 6: ERAD inhibition and ER stress triggered by Htt96Q can be compensated by overexpression of p97/VCP. ( a ) Induction of eIF2α phosphorylation after 24 h of Htt96Q expression is strongly inhibited by coexpression of p97/VCP. (* P -value=0.02, Student’s t -test (unpaired, two-tailed)). ( b ) Accumulation of H2a caused by Htt96Q expression is strongly reduced by coexpression of p97/VCP. P97/VCP has only a minor, non-significant effect in reducing the Htt96Q fraction in insoluble aggregates. Values were corrected by the anti-β-tubulin signal as a loading control. (** P -value<0.01, *** P -value=0.00006, Student’s t -test (unpaired, two-tailed)). ( c ) Inhibition of H2a degradation on expression of Htt96Q is cancelled by overexpression of p97/VCP. Experiment similar to that in Fig. 1b but in HEK 293 cells with and without coexpression of p97. The graph shows percent of H2a in the chase relative to pulse (100%). Where indicated, p97 overexpression was done using 6xHis-tagged p97/VCP in all cases. All graphs in this figure are averages of three experiments±s.e. Full size image ERAD substrate accumulation before visible Htt aggregates The above experiments showed the average response of a heterogeneous cell population. To achieve better resolution, we analysed individual cells by time-lapse microscopy. As the fluorescent signal of the XBP1-venus reporter was too weak for this type of experiment, we coexpressed H2a-GFP together with TEToff-regulated Htt96Q fused to fluorescent mCherry protein (Htt96Q-Cherry) in striatal cells. Expression of the latter was shut off by addition of Dox 2–3 h before the start of the experiment to reduce the fraction of newly made monomeric Htt96Q-Cherry ( Fig. 7a ) and focus on the transition from oligomers to visible inclusions of aggregated protein. Htt96Q-Cherry appeared in a diffuse cytosolic and nuclear pattern until a certain time after transfection, when visible aggregates appeared and very rapidly recruited almost all of the cellular protein, in many cells in a matter of minutes ( Fig. 7b,c and Supplementary Movies 1 and 2 ). The rapid sequestration of most Htt96Q-Cherry into visible aggregates also occurred in cells without shut-off of Htt synthesis by Dox addition ( Supplementary Movie 3 ). Coexpressed H2a-GFP accumulated gradually in the juxtanuclear ERQC, starting 60–120 min before the appearance of visible Htt96Q-Cherry aggregates ( Fig. 7b,c and Supplementary Movies 1 and 2 ). H2a-GFP accumulation in cells without shut-off of Htt synthesis showed a similar response ( Supplementary Movie 3 ). H2a-GFP accumulation in the cells was in response to the pre-aggregation process of Htt96Q-Cherry and did not occur in the absence of visible aggregation ( Fig. 8c and Supplementary Movie 4 ). Cellular accumulation of H2a-GFP in general and in the ERQC in particular continued but in some cells at a slower pace after appearance of visible aggregates ( Figs 7c and 8a ). 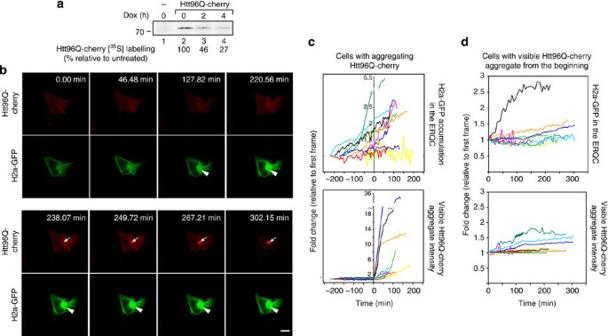Figure 7: Progressive ERAD substrate accumulation in the ERQC before appearance of visible Htt aggregates. (a) The drop in Htt synthesis using TEToff regulation was verified by metabolic labelling for 30 min with [35S]-(Met+Cys) and IP of Htt96Q-Cherry expressed in STHdhQ7/7cells following incubation with Dox for the indicated periods. (b) Live imaging of a representative STHdhQ7/7cell expressing Htt96Q-Cherry and H2a-GFP, after shut-off of Htt96Q-Cherry synthesis. Arrow: appearance of a visible large Htt96Q-Cherry aggregate. Arrowhead: H2a-GFP juxtanuclear accumulation. Scale bar, 10 μm. The corresponding movie can be seen inSupplementary Movie 1. (c) H2a-GFP accumulation in the ERQC relative to Htt96Q-Cherry aggregation (from seven independent experiments). Zero: first appearance of a visible Htt96Q-Cherry aggregate. Each line colour represents the same individual cell in both graphs. (d) As inc, but in cells with the presence of visible Htt96Q-Cherry aggregates and H2a-GFP accumulation from the beginning of the observation, (from six independent experiments). Figure 7: Progressive ERAD substrate accumulation in the ERQC before appearance of visible Htt aggregates. ( a ) The drop in Htt synthesis using TEToff regulation was verified by metabolic labelling for 30 min with [ 35 S]-(Met+Cys) and IP of Htt96Q-Cherry expressed in ST Hdh Q7/7 cells following incubation with Dox for the indicated periods. ( b ) Live imaging of a representative ST Hdh Q7/7 cell expressing Htt96Q-Cherry and H2a-GFP, after shut-off of Htt96Q-Cherry synthesis. Arrow: appearance of a visible large Htt96Q-Cherry aggregate. Arrowhead: H2a-GFP juxtanuclear accumulation. Scale bar, 10 μm. The corresponding movie can be seen in Supplementary Movie 1 . ( c ) H2a-GFP accumulation in the ERQC relative to Htt96Q-Cherry aggregation (from seven independent experiments). Zero: first appearance of a visible Htt96Q-Cherry aggregate. Each line colour represents the same individual cell in both graphs. ( d ) As in c , but in cells with the presence of visible Htt96Q-Cherry aggregates and H2a-GFP accumulation from the beginning of the observation, (from six independent experiments). 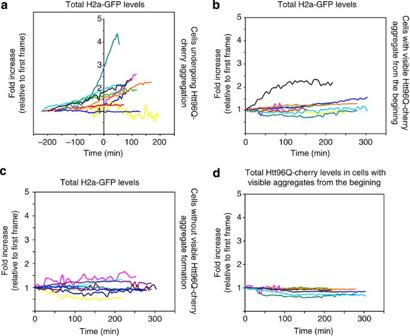Figure 8: Total H2a-GFP and Htt96Q-Cherry levels in time-lapse experiments. (a–c) The graphs summarize total H2a-GFP levels in the cells with aggregating Htt96Q-Cherry (a), with visible Htt96Q-Cherry aggregates from the beginning (b) or without the appearance of large Htt96Q-Cherry aggregates (c). (d) Total Htt96Q-Cherry levels remained stable throughout the experiment in the Dox-treated cells. Full size image Figure 8: Total H2a-GFP and Htt96Q-Cherry levels in time-lapse experiments. ( a – c ) The graphs summarize total H2a-GFP levels in the cells with aggregating Htt96Q-Cherry ( a ), with visible Htt96Q-Cherry aggregates from the beginning ( b ) or without the appearance of large Htt96Q-Cherry aggregates ( c ). ( d ) Total Htt96Q-Cherry levels remained stable throughout the experiment in the Dox-treated cells. Full size image ERAD substrate does not accumulate with Htt aggregate growth Accumulation of H2a-GFP did not continue, or became very slow, sometime after the appearance of visible aggregates of Htt96Q-Cherry (except for one of the monitored cells in one experiment; Figs 7d and 8b ). A sharp contrast between the accumulation of the ERAD substrate at pre-aggregation stages of Htt96Q and a lack of accumulation in response to large aggregate concentration can better be observed in Fig. 9 , where we have plotted the accumulation of H2a-GFP in the ERQC versus the fraction of Htt96Q-Cherry in visible aggregates at each time point. For cells where Htt96Q was in the process of aggregation ( Fig. 9a ), there was a robust increase in H2a-GFP accumulation before visible aggregation but no correlation afterwards with the increase in the fraction of visibly aggregated Htt. Thus, the ERAD substrate does not accumulate in correlation with the concentration of visible aggregates. For cells where Htt96Q was already visibly aggregated from the start of the experiment ( Fig. 9b ), there was very little increase or decrease in H2a accumulation. This suggests that these cells are in a metastable state where increase in ER stress is arrested but the pre-existing stress is not reduced in the time frame of the experiment. 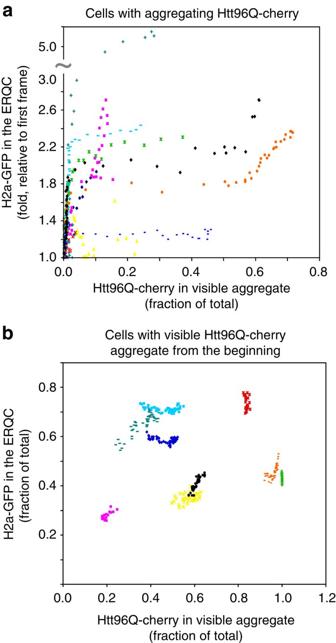Figure 9: Lack of dependence of ERAD substrate accumulation on Htt concentration in visible aggregates (a,b). Relationship between H2a-GFP accumulation and Htt96Q-Cherry aggregation fromFig. 7. Each colour represents the same individual cell. H2a-GFP concentration sharply increases before the appearance of visible Htt96Q-Cherry aggregates, with little or no increase in response to aggregate growth (a). Sometime after visible Htt96Q-Cherry aggregate appearance (b), there is very little increase in H2a-GFP accumulation, and no correlation between H2a-GFP and Htt96Q-Cherry concentrations. Figure 9b also shows that there is no correlation between the fraction of Htt96Q in visible aggregates and the degree of H2a-GFP accumulation. Again, this suggests that the ERAD substrate does not accumulate in correlation with the concentration of visible aggregates. There was also very little increase in the fraction of Htt96Q in visible aggregates, each cell having reached an equilibrium at very different concentrations of the protein as a fraction of total ( Fig. 9b ). Total Htt96Q levels remained constant during this time course ( Fig. 8d ). Figure 9: Lack of dependence of ERAD substrate accumulation on Htt concentration in visible aggregates ( a , b ). Relationship between H2a-GFP accumulation and Htt96Q-Cherry aggregation from Fig. 7 . Each colour represents the same individual cell. H2a-GFP concentration sharply increases before the appearance of visible Htt96Q-Cherry aggregates, with little or no increase in response to aggregate growth ( a ). Sometime after visible Htt96Q-Cherry aggregate appearance ( b ), there is very little increase in H2a-GFP accumulation, and no correlation between H2a-GFP and Htt96Q-Cherry concentrations. Full size image The sudden aggregation of polyQ-expanded Htt in single cells, occurring at different Htt concentrations (as a fraction of total), suggests that the aggregation requires a stochastic seeding event, independently of Htt96Q concentration in the cell. After visible aggregates appear, each cell rapidly reaches a certain level of Htt concentration and ERAD substrate accumulation, which are not interdependent ( Fig. 9b ). Each cell is in its own situation or ‘space’ of protein homoeostasis, which probably depends on its individual buffering capacity [25] . ERAD substrate accumulation and the consequent ER stress are not dependent on the presence and concentration of large visible aggregates but arise when Htt is in a monomeric or oligomeric state ( Figs 5 , 6 , 7 , 8 , 9 ). The ER stress generated correlates best with the presence of oligomeric species, the advent of which may be triggered by a proteolytic processing event of Htt ( Fig. 5 ). ER stress is only slowly reduced after shutting off the synthesis of new Htt, even when insoluble aggregates have already formed ( Fig. 5 ). The accumulation of the ERAD substrate caused by oligomeric Htt species is consistent with the reported inhibition of the UPS before Htt aggregation using cytosolic proteasome substrates [17] , [18] , although these have sometimes been observed to accumulate only after visible aggregation [26] , perhaps reflecting the buffering capacity of the cell type studied. We propose the following model to explain the mechanism of ER stress caused by the mutant Htt oligomers ( Fig. 10 ). Monomers of mutant Htt exon 1 can polymerize into large aggregates or organize into different types of oligomers with differential toxicity [27] . ‘Toxic’ oligomers, of a defined structure or size, are generated some time before the appearance of visible aggregates. These oligomers interact with p97/VCP and possibly with other chaperones and components of the ubiquitin-proteasome machinery, transcription factors and so on [3] , depleting them with time and impairing their normal function. These types of oligomers may represent ‘kinetically trapped species’ converting only slowly to large aggregates. In contrast, once formed, large aggregates would rapidly recruit monomers (and possibly also non-toxic oligomers) and their sequestration would prevent them from serving as a possible source of toxic oligomers. The time-lapse experiments suggest that the large aggregates are very efficient in this sequestration, depleting rapidly most newly synthesized species in many cells. The stress levels do not increase in response to the growth of large aggregates, but they are reduced, albeit only gradually, as the conversion of toxic oligomers into large aggregates is slow. In the long term, the toxic species are slowly recruited into large aggregates, or may be degraded, which enables some alleviation of the stress. However, this process seems to be kinetically inefficient, and pro-apoptotic mechanisms that derive from prolonged ER stress [22] are likely activated in most cells. 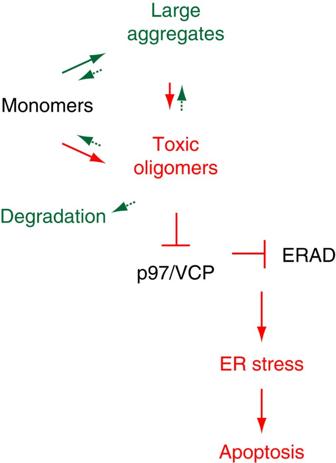Figure 10: A proposed model for Htt toxicity. Green indicates a cell-protective pathway and red a toxic one. Htt monomers can be quickly captured into large insoluble aggregates or converted to toxic oligomers. Toxic oligomers, which are inefficiently converted to non-toxic species or degraded, sequester p97/VCP, interfering with ERAD and leading to ER stress and in the long term to apoptosis. Figure 10: A proposed model for Htt toxicity. Green indicates a cell-protective pathway and red a toxic one. Htt monomers can be quickly captured into large insoluble aggregates or converted to toxic oligomers. Toxic oligomers, which are inefficiently converted to non-toxic species or degraded, sequester p97/VCP, interfering with ERAD and leading to ER stress and in the long term to apoptosis. Full size image In conclusion, the onset of ER stress, which arises as a consequence of ERAD inhibition, correlates with the formation of Htt oligomers and precedes the formation of visible inclusions. This mechanism might be shared by other protein misfolding diseases, for example, Alzheimer’s and Parkinson’s, for which there is evidence for the involvement of oligomeric states [28] , [29] , [30] . P97 depletion appears to be a major factor in the process of ER stress induction by Htt oligomers, and possibly also in other diseases involving protein aggregation, consistent with the fact that p97 mutations can cause or exacerbate neurodegeneration [31] . Materials Promix cell labelling mix ([ 35 S]Met plus [ 35 S]Cys), >1,000 Ci mmol −1 was from PerkinElmer (Boston, MA). Ni-NTA agarose was from Qiagen (Valencia, CA) and protein A-Sepharose from Repligen (Needham, MA). MG-132, tunicamycin, Dox, DMEM Cys/Met-free and other common reagents were from Sigma. Lactacystin was from Calbiochem. Plasmids and constructs H2a subcloned in pCDNA1 and uncleavable H2aG78R fused through its carboxy terminus with the linker SGGGGS to monomeric RFP (H2a-RFP) expressing vectors were used before [19] , [21] . H2a-GFP was constructed by insertion of H2aG78R followed by the SGGGGS linker into the pEGFP-N1 vector (Clontech) using Eco RI and Bam HI restriction sites. Myc-tagged exon 1 Htt20Q and Htt96Q are subcloned in pTREhygro vectors controlled by pTet-Off regulatory plasmid [3] . Htt96Q-Cherry was produced by PCR in two steps. First, the stop codon was converted to glycine using 5′-ATATTAGCGGCCGCATTATGTGTGAAC-3′ and 5′-ATATTAGTCGACTCCCGGTCGGTGCAGCGGCTC-3′ primers and the product replaced the original Htt96Q in Not 1 and Sal 1 restriction sites. Second, mCherry was amplified using 5′-ATATTAGTCGACAGCGGAGGTGGAGGTAGCATGGTGAGCAAGGGCGAGGAG-3′ and 5′-AATATAGATATCCTACTTGTACAGCTCGTCCATG-3′ primers and subcloned downstream to Htt96Q using Sal 1 and Eco RV restriction sites. OS-9.1 and OS-9.2 are S-tagged in their amino terminus, with the signal sequence from bovine preprolactin followed by the S-tag and in frame fusion without the endogenous signal sequence [32] . F- XBP1D DBD- venus cloned in pCAX (XBP1-venus) [23] , 6xHis-tagged p97/VCP wild type in pcDNA3 and BiP-GFP were kind gifts of Masayuki Miura (Brain Science Institute, Saitama, Japan), Linda M. Hendershot (St. Jude Children’s Research Hospital, Memphis) and Erik Snapp (Albert Einstein College of Medicine, NY), respectively. Antibodies Rabbit polyclonal anti-H2a C-terminal and anti-N-terminal antibodies were the ones used in earlier studies [20] at 1:1,000 for immunoblot (IB) and 1:100 for immunoprecipitation (IP). Other rabbit antibodies were as follows; anti-calnexin (1:500) from Sigma (C4731), anti-phospho-eIF2α (Ser51) (1:500) from Cell Signaling (3597), anti-GADD34 (1:2,000) was a kind gift of David Ron and anti-BiP (1:1,000) was a kind gift of Linda M. Hendershot. Mouse monoclonal antibodies were as follows; anti-c-Myc (1:1,000 IB, 1:100 IP, 1:300 immunofluorescence) from Santa Cruz (SC-40), anti-β-tubulin (1:1000) from Sigma (T4026), anti-GAPDH (1:8,000) from Chemicon International MAB374, anti-ATF6 (1:50) from Abnova (MAB0082), anti-His-tag (1:2,000) from Aviva Systems Biology (OAEA00010) and anti-S tag (1:250) from Novagen (71549). Goat anti-mouse IgG conjugated to Cy2 (1:250) (205-225-108), goat anti-rabbit IgG-Cy3 (1:300) (111-165-144), and goat anti-rabbit (111-035-144) and anti-mouse IgG conjugated to horseradish peroxidase (115-035-166) (1:5,000) were from Jackson Labs. Cell culture and transfections HEK 293, NIH 3T3 and N2a cells (ATCC) were grown in DMEM plus 10% FCS at 37 °C under 5% CO 2 . ST Hdh Q7/7 and ST Hdh Q111/111 cells were a kind gift of Marcy E. MacDonald and grown at 33 °C in DMEM plus 10% FCS [33] . Transient transfections of NIH 3T3, N2a and ST Hdh Q7/7 cells were performed using an MP-100 Microporator (Digital Bio), according to the manufacturer’s protocols. HEK 293 cells were transfected according to calcium phosphate method. Htt96Q or Htt20Q were cotransfected with tetracycline-controlled pTet-Off regulatory plasmid in 1:3 ratio in all cases. Metabolic labelling and IP Subconfluent (90%) cell monolayers in 60-mm dishes were labelled with 200 μCi per 0.5 ml of [ 35 S]Cys or [ 35 S]Cys+Met mix as indicated, lysed and immunoprecipitated with anti-H2 antibodies, as described in ref. 20 . Briefly, cells were rinsed and preincubated for 30 min at 37 °C with Cys-free or Cys and Met-free DMEM plus 10% dialyzed calf serum. They were then pulse labelled in the same medium containing [ 35 S]Cys or [ 35 S]Cys+Met for 30 min. Cells were then rinsed and chased for different periods of time with normal DMEM plus 10% FCS. After rinsing with PBS, cells were lysed in 1% Triton X-100 and 0.5% sodium deoxycholate in PBS with protease inhibitors. IPs from cell lysates were performed with rabbit anti-H2a C-terminal antibody and protein A-Sepharose or mouse anti-myc and goat anti-mouse IgG-agarose for myc-tagged Htt at 4 °C for 16 h. The beads were then washed three times with diluted lysis buffer and the proteins were eluted with sample buffer containing 1% SDS and 5% β-mercaptoethanol at 100 °C for 5 min. SDS–PAGE and quantitation SDS–polyacrylamide gel electrophoresis (PAGE) was performed on 12% Laemmli gels. Gels with radioactive samples were analysed by fluorography using 20% 2,5-diphenyloxazole and exposed to Biomax MR film from Kodak (Vancouver, BC). Quantitation was performed in a Fujifilm FLA 5100 phosphorimager (Japan). Detection of 6xHis-tagged P97/VCP Transfected cells were lysed with 1% Triton X-100, 50 mM NaH 2 PO 4 , 300 mM NaCl and 10 mM imidazole at pH 8.0. The lysates were centrifuged and the nuclei and cell debris discarded. The supernatants were rotated gently with Ni-NTA agarose for 2–3 h at 4 °C. The beads were washed three times with wash buffer (same as lysis buffer, but with 20 mM imidazole) and proteins were eluted with elution buffer (same as the lysis buffer, but with 250 mM imidazole) for 1 min on ice. The eluate was collected, boiled with sample buffer and run on SDS–PAGE as above. His-tagged P97/VCP was detected by IB using mouse anti-His-tag antibody. Treatments and immunoblotting Cells were treated with 5 μg ml −1 tunicamycin for 13–16 h or with 10 μg ml −1 for 2 h as indicated. A final concentration of 1 μg ml −1 of Dox was used in all the experiments where indicated. Cells were lysed with PBS containing 1% Triton X-100, 0.5% sodium deoxycholate with protease inhibitors and centrifuged to pellet insoluble aggregates, debris and nuclei. Sodium fluoride (10 mM) and 10 mM β-glycerolphosphate were added to the lysis buffer to inhibit phosphatases for detection of phosphorylated proteins. Treatment with lactacystin was performed for 3–5 h at the final concentration of 17 μM. Supernatants were separated from pellets and incubated in loading buffer for 5 min at 100 °C, pellets were incubated for 10 min. For IB, after SDS–PAGE and transfer to nitrocellulose membrane, blocking was done in 5% low-fat milk and 0.1% Tween-20 in PBS for 1 h. Incubation with the primary antibody was overnight at 4 °C and after three washes in 0.1% Tween-20 in PBS, incubation with the appropriate secondary antibody was for 1 h at room temperature. After washing, enhanced chemiluminescence assay was performed and the membrane was exposed and quantified in a Bio-Rad ChemiDocXRS Imaging System (Bio-Rad, Hercules, CA) [32] . Images of full-length blots for all figures are provided in Supplementary Fig. S1 . RT–PCR Total-cell RNA was extracted using TRIzol reagent (Invitrogen). PCR was done using ReddyMix (ABgene, Epsom, UK) [32] . Reverse transcription (RT) was performed with a VersoTM cDNA kit (Thermo Fisher Scientific, Barrington, IL) using a mixture of random hexamer and anchored oligo-dT primers. An aliquot (10%) of the RT product was used for PCR. Primers for BiP amplification were 5′-GCAGGACATCAAGTTCTTGCC-3′ and 5′-CCGGAGTTTCTGCACAGCTC-3′. Primers for spliced XBP1 amplification were 5′-TCTGCTGAGTCCGCAGCAG-3′ and 5′-GAAAAGGGAGGCTGGTAAGGAAC-3′, and for GAPDH were 5′-CTTTTAACTCTGGTAAAGTGG-3′ and 5′-TTTTGGCTCCCCCCTGCAAAT-3′ (ref. 32 ). Glycerol gradient fractionation Cells expressing Htt96Q were lysed in 1% Triton/PBS with protease inhibitors and centrifuged to separate insoluble aggregates (pellet) from soluble proteins (supernatant). The supernatants were loaded on top of a glycerol gradient (8.5–35%). Glycerol solutions were prepared in 0.1% Triton/PBS. The gradients were ultracentrifuged at 38,000 r.p.m. (~247,000 g , Beckman SW41 rotor) for 16 h at 4 °C. Markers of known molecular weight including BSA, aldolase, catalase, ferritin and thyroglobulin were ultracentrifuged in parallel. Twelve fractions were collected from gradient top to bottom (light to heavy), precipitated by trichloroacetic acid and subjected to immunoblotting. Immunofluorescence Cells grown for 24 h after transfection on coverslips in 24-well plates were fixed with 3% paraformaldehyde, followed by blocking with 50 mM glycine in PBS and normal goat IgG in PBS/2% BSA. The cells were incubated with primary antibodies for 1 h, washed and incubated for 30 min with secondary antibodies, followed by washes. Nuclei were stained with 4',6-diamidino-2-phenylindole. The samples were observed in a Leica fluorescence microscope. Live cell imaging Cells were grown on 25 mm coverslips in six-well plates for 24 h after transfection. Dox (1 μg ml −1 ) was added 2–3 h before the observation and remained in the medium during the imaging, if not indicated otherwise. The coverslips were incubated in a temperature-controlled chamber at 37 °C under 5% CO 2 and observed using a Zeiss laser scanning confocal microscope (LSM 510 Meta; Carl Zeiss, Jena, Germany) under the command of ZEN software. Lasers of 488 and 561 nm were used. The acquired images were analysed in ImageJ. Statistical analysis Data are expressed as means±s.e. Student’s t -test (unpaired, two-tailed) was used to compare the two groups, and the P -value was calculated in GraphPad Prism 5 (GraphPad Software). P ≤0.05 was considered as statistically significant. How to cite this article: Leitman, J. et al. Soluble forms of polyQ-expanded huntingtin rather than large aggregates cause endoplasmic reticulum stress. Nat. Commun. 4:2753 doi: 10.1038/ncomms3753 (2013).